The structural basis for the negative regulation of thioredoxin by thioredoxin-interacting protein The redox-dependent inhibition of thioredoxin (TRX) by thioredoxin-interacting protein (TXNIP) plays a pivotal role in various cancers and metabolic syndromes. However, the molecular mechanism of this regulation is largely unknown. Here, we present the crystal structure of the TRX–TXNIP complex and demonstrate that the inhibition of TRX by TXNIP is mediated by an intermolecular disulphide interaction resulting from a novel disulphide bond-switching mechanism. Upon binding to TRX, TXNIP undergoes a structural rearrangement that involves switching of a head-to-tail interprotomer Cys63-Cys247 disulphide between TXNIP molecules to an interdomain Cys63-Cys190 disulphide, and the formation of a de novo intermolecular TXNIP Cys247-TRX Cys32 disulphide. This disulphide-switching event unexpectedly results in a domain arrangement of TXNIP that is entirely different from those of other arrestin family proteins. We further show that the intermolecular disulphide bond between TRX and TXNIP dissociates in the presence of high concentrations of reactive oxygen species. This study provides insight into TRX and TXNIP-dependent cellular regulation. Human thioredoxin (TRX) reduces disulphides on targeted proteins, and in that role it is crucial in modulating intra- and extracellular signalling pathways by inducing a number of transcription factors such as Ref-1, p53, NF-κB, and AP-1 that regulate various aspects of cell growth and survival [1] . TRX is upregulated in a variety of human tumours, including lung, pancreatic, colon, gastric, and breast cancer, although the molecular mechanisms by which TRX augments tumorigenesis are unclear [2] . Upregulation of TRX is associated with inhibition of apoptosis, promotion of tumour cell proliferation, aggressive tumour growth, and reduced patient survival [3] , [4] . TRX directly binds to and inhibits the proapoptotic protein apoptosis signal-regulating kinase-1 (ref. 5 ) and the tumour-suppressor PTEN, a protein that hydrolyses membrane phosphatidylinositol-3-phosphates and attenuates the activity of the phosphatidylinositol-3-kinase/Akt cell survival pathway [6] in a redox-dependent manner. Due to these cell growth-promoting effects and its ability to inhibit apoptosis, TRX has emerged as an attractive molecular target for new anticancer drugs [7] , [8] . Thioredoxin-interacting protein (TXNIP), also known as vitamin D 3 -upregulated protein-1 or TRX-binding protein-2, is an endogenous inhibitor of TRX [9] , [10] . Inhibition of TRX by TXNIP reduces the ability of TRX to interact with a number of other cellular molecules, thereby affecting cell signalling; hence, TXNIP has emerged as an important element in the pathogenesis of many cancers and metabolic diseases [11] , [12] . TXNIP has a critical function in cell growth and acts as a tumour suppressor [13] . In contrast to TRX, which is upregulated in many cancers [2] , TXNIP is strongly downregulated in a variety of tumour tissues and cell lines [14] , [15] , [16] , [17] . TXNIP-deficient mice have an increased incidence of hepatocellular carcinoma [18] , while xenotransplants of HEp-2 cells overexpressing TXNIP display significantly reduced tumorigenesis [19] . These tumour-suppressing functions of TXNIP are due, in many cases, to its inhibition of TRX. TXNIP co-localizes with and reduces the activity of TRX in Jurkat T cells treated with the tumour-suppressor lipid ceramide, leading to dissociation of TRX from apoptosis signal-regulating kinase-1, ER stress, phosphorylation of p38 and JNK, and subsequent cellular apoptosis [20] . Similar TXNIP activity was observed in an ovarian cancer cell line treated with a synthetic retinoid [21] . Furthermore, the histone methyltransferase inhibitor 3-deazaneplanocin A upregulates TXNIP and inhibits TRX in cancer cell lines, thereby increasing reactive oxygen species (ROS) levels and promoting apoptosis [22] . Similarly, treatment of tumour cells with suberoylanilide hydroxamic acid, a potent inhibitor of histone deacetylases, induces TXNIP expression, reduces TRX levels, and causes growth arrest, differentiation and/or apoptosis [17] . TXNIP is also a metabolic control protein, although it is unclear whether it acts in this context by inhibiting TRX [23] , [24] , [25] , [26] . TXNIP expression is strongly correlated with extracellular glucose levels. Glucose stimulates TXNIP transcription through a carbohydrate-response element in the TXNIP promoter [27] and its association with max-like protein X and MondoA transcription factors [28] . Elevated levels of TXNIP lead to a reduction in the number of pancreatic β-cells, insulin secretion, and peripheral glucose uptake [24] , [28] . By contrast, TXNIP deficiency protects against β-cell apoptosis, enhances insulin sensitivity, and counteracts hyperglycaemia and glucose intolerance [29] , [30] . Although the role of TXNIP in glucose metabolism may not require interaction with TRX, TXNIP does regulate other metabolic functions via this interaction. Binding to TRX promotes TXNIP stability, which can block adipocyte differentiation [31] . In response to increased ROS levels, TXNIP is released from TRX and binds to the inflammasome protein NLRP3, which may link metabolism with the innate immune response [32] . Considerable efforts have been made to understand the molecular mechanism of the inhibition of TRX by TXNIP. TXNIP belongs to the α-arrestin family, which also includes the arrestin domain-containing proteins 1–5 in humans; these proteins contain PPxY motifs in the C-terminal region [33] . However, TXNIP is the only α-arrestin family member that binds to and negatively regulates TRX. Patwari et al. demonstrated that the Cys32 residue of TRX and the Cys247 residue of TXNIP form a stable mixed disulphide and proposed that TXNIP contains an intramolecular disulphide bond between Cys63 and Cys247 that allows it to interact with TRX [34] . Notably, TXNIP contains 11 cysteines, a uniquely large number, while TRX contains five. Although important insights into the interaction between TRX and TXNIP have been made, the exact molecular mechanism by which TXNIP interacts with and negatively regulates TRX has not yet been elucidated. Several essential questions still remain: because TXNIP has a distinct ability to regulate TRX, should it be classified in the α-arrestin family? How can an intramolecular disulphide between Cys63 and Cys247 in TXNIP be formed in a topological sense? What is the role of TXNIP Cys63 in the interaction with TRX? What roles do other cysteines in TXNIP play in the interaction with TRX? What molecular mechanism does TXNIP employ to regulate TRX? To answer these questions, we performed structural studies of the interaction between TRX and TXNIP. Here we report the crystal structures of the heterodimeric TRX–TXNIP complex and the N-terminal domain of TXNIP. In combination with co-immunoprecipitation, NMR, and biochemical data, the structures suggest that the interaction between TRX and TXNIP is regulated by a redox-dependent disulphide bond-switching mechanism. Molecular architecture of the TRX–TXNIP complex Repeated attempts to overexpress recombinant full-length TXNIP as a soluble protein failed; however, the complex of TRX and T–TXNIP (amino acids 3–317) was soluble ( Fig. 1a ). Because TRX and TXNIP are redox proteins and their properties make them difficult to handle in vitro , we mutated TRX Cys35 to Ala to prevent further reactions after interaction of the proteins. Cysteine mutations in T–TXNIP were also generated to prevent non-specific covalent oligomerization and to enable the generation of crystals suitable for X-ray diffraction. Two mutant complexes, TRX(C35A)–T–TXNIP(C120S/C170S/C205S/C267S) (hereafter referred to as Com1) and TRX(C35A)–T–TXNIP(C170S/C205S/C267S) (hereafter referred to as Com2), were crystallized to X-ray diffraction quality and their structures were determined using the multiple anomalous wavelength dispersion method, together with the molecular replacement (MR) method. The structures of Com1 and Com2 ( Fig. 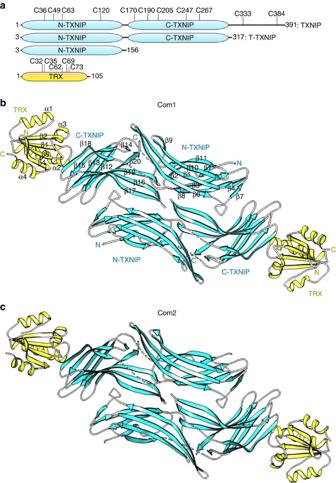Figure 1: Overall structure of the heterodimeric complex of TRX and TXNIP in the asymmetric unit. (a) Schematic representation of the TXNIP (cyan) and TRX (yellow) constructs used in this study, showing the locations of the cysteines. (b,c) Ribbon representations of the structures of the TRX(C35A)–T–TXNIP(C120S/C170S/C205S/C267S) complex (referred to as Com1) (b) and the TRX(C35A)–T–TXNIP(C170S/C205S/C267S) complex (referred to as Com2) (c). The structures of Com1 and Com2 were determined at resolutions of 2.0 Å and 2.7 Å, respectively. There are two heterodimeric complexes of TRX and TXNIP in the asymmetric unit. The β-sheets and disordered regions of TXNIP are shown in cyan and by white dashed lines, respectively. The α-helices and β-sheets of TRX are shown in yellow. The N-terminal TXNIP (N-TXNIP) and C-terminal TXNIP (C-TXNIP) domains are indicated. 1b,c ) were refined to resolutions of 2.0 Å and 2.7 Å, respectively ( Table 1 ). The abilities of mutated TXNIP and T–TXNIP to bind TRX ( Supplementary Fig. S1a,b ) and inhibit its activity ( Supplementary Fig. S1c ) were comparable to that of native TXNIP. Therefore, the crystal structures of Com1 and Com2 are representative of interactions between TRX and TXNIP. Figure 1: Overall structure of the heterodimeric complex of TRX and TXNIP in the asymmetric unit. ( a ) Schematic representation of the TXNIP (cyan) and TRX (yellow) constructs used in this study, showing the locations of the cysteines. ( b , c ) Ribbon representations of the structures of the TRX(C35A)–T–TXNIP(C120S/C170S/C205S/C267S) complex (referred to as Com1) ( b ) and the TRX(C35A)–T–TXNIP(C170S/C205S/C267S) complex (referred to as Com2) ( c ). The structures of Com1 and Com2 were determined at resolutions of 2.0 Å and 2.7 Å, respectively. There are two heterodimeric complexes of TRX and TXNIP in the asymmetric unit. The β-sheets and disordered regions of TXNIP are shown in cyan and by white dashed lines, respectively. The α-helices and β-sheets of TRX are shown in yellow. The N-terminal TXNIP (N-TXNIP) and C-terminal TXNIP (C-TXNIP) domains are indicated. Full size image Table 1 Data collection and refinement statistics for complex structures. Full size table The structures of Com1 and Com2 are essentially identical; each structure contains two heterodimeric complexes of TRX and T–TXNIP in an asymmetric unit, with a large interface between the two T–TXNIP molecules ( Fig. 1b,c ). However, size-exclusion chromatography revealed that all of the complexes, including the native complex, exist as single heterodimeric species in solution ( Supplementary Fig. S2 ); therefore, the interfaces between the T–TXNIP molecules in the crystal structures merely constitute large crystal contacts. Since the two structures are essentially identical and the TRX and T–TXNIP complex exists as a single heterodimeric species in solution, the T–TXNIP (chain C) and TRX (chain D) complex ( Fig. 1b ) of Com1 was chosen as a representative structure and is hereafter referred to unless otherwise specified. The final structure of the heterodimeric complex contains residues 8–299 of the expressed protein, residues 3–317 of T–TXNIP and full-length TRX. Residues 148–153 and 260–265 of T–TXNIP are not included in the final model because they are not visible in the electron density map; these regions are presumably very flexible. T–TXNIP is composed entirely of β-strands that form two deeply curved β-sandwich domains: an N-terminal domain (N-TXNIP) consists of strands β1 to β11 (residues 8–147) and a C-terminal domain (C-TXNIP) consists of strands β12 to β20 (residues 154–299) ( Figs 1b and 2a ). The protein folds into an elongated S-shaped domain arrangement with pseudo-2-fold symmetry in which C-TXNIP is inverted relative to N-TXNIP. The two domains can be superimposed with a root-mean-square deviation (RMSD) of 1.88 for 60 Cα atoms ( Supplementary Fig. S3 ). Although the domain arrangement of T–TXNIP in complex with TRX is completely different to that of all other arrestin structures reported (which have ω-shaped domains), the overall structure of T–TXNIP is similar to that of proteins in the arrestin superfamily, including mouse vacuolar protein sorting-associated protein 26B (mVPS26B; Protein Data Bank accession code 3LH8) ( Supplementary Fig. S4 ) [35] . Therefore, tandem T–TXNIP, comprising the N-TXNIP and C-TXNIP domains, could not be superimposed onto the mVPS26B structure ( Fig. 2b ), while the individual N-TXNIP (RMSD=1.33 for 82 Cα atoms; Z=12.3) and C-TXNIP (RMSD=1.42 for 84 Cα atoms; Z=12.5) domains could be superimposed onto each N-mVPS26B and C-mVPS26B domain, respectively ( Fig. 2c ). The structural analysis also revealed that T–TXNIP is electrically polarized ( Fig. 2d ). In particular, the inside section of the curved β-sandwich of the C-TXNIP domain contains a prominent basic region, while N-TXNIP has a negative electrostatic potential. 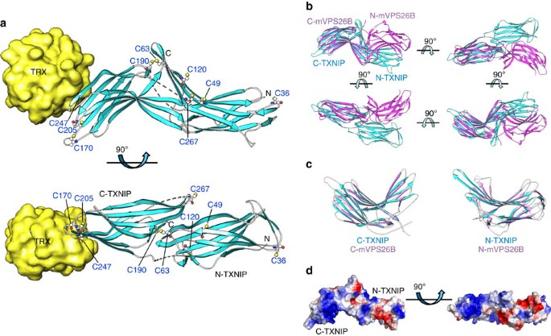Figure 2: Representative structure of the TRX and TXNIP complex and structural comparison between TXNIP and arrestin. (a) TRX interacts exclusively with C-TXNIP in the complex structure. The β-strands and disordered regions of TXNIP are shown in cyan and as grey dashed lines, respectively. The cysteines in TXNIP are displayed as white carbon atoms. Cys63 is located 39 Å from Cys247 and 14.1 Å from Cys120. (b) TRX-bound TXNIP (cyan) superimposed onto mVPS26B (magenta) based on the C-terminal domains. The disordered regions of TXNIP and mVPS26B are shown as dashed cyan and magenta lines, respectively. (c) Superimposition of N-TXNIP and C-TXNIP (cyan) onto N-mVPS26B and C-mVPS26B (magenta). The disordered region of C-TXNIP is shown as a dashed white line. (d) The electrostatic surface potential of TXNIP shows a highly basic C-terminal domain and a relatively negative electrostatic N-terminal domain. Figure 2: Representative structure of the TRX and TXNIP complex and structural comparison between TXNIP and arrestin. ( a ) TRX interacts exclusively with C-TXNIP in the complex structure. The β-strands and disordered regions of TXNIP are shown in cyan and as grey dashed lines, respectively. The cysteines in TXNIP are displayed as white carbon atoms. Cys63 is located 39 Å from Cys247 and 14.1 Å from Cys120. ( b ) TRX-bound TXNIP (cyan) superimposed onto mVPS26B (magenta) based on the C-terminal domains. The disordered regions of TXNIP and mVPS26B are shown as dashed cyan and magenta lines, respectively. ( c ) Superimposition of N-TXNIP and C-TXNIP (cyan) onto N-mVPS26B and C-mVPS26B (magenta). The disordered region of C-TXNIP is shown as a dashed white line. ( d ) The electrostatic surface potential of TXNIP shows a highly basic C-terminal domain and a relatively negative electrostatic N-terminal domain. Full size image TRX interacts exclusively with C-TXNIP in the complex structure. No significant structural changes were observed in the structure of TRX complexed with T–TXNIP compared with the previously reported free TRX structure ( Supplementary Fig. S5 ) [36] . Detailed characterization of the TRX–TXNIP interaction Cys247 in TXNIP is required for the interaction with Cys32 in TRX [34] . The intermolecular disulphide bond between these residues is located in the centre of the interaction interface between the two proteins ( Fig. 3a,b ). The β18 strand of T–TXNIP, in combination with β15, is a critical component of the interaction, and the overall conformation of bound β18 is extended and follows the cleft formed by residues in the active site of TRX. Intermolecular backbone–backbone interactions between TRX and residues in the β18 strand of T–TXNIP (TRX Ala92 and T–TXNIP Gly245, and TRX Met74 and T–TXNIP Cys247) stabilize the interaction ( Fig. 3c ). In addition, intermolecular hydrogen bonds and hydrophobic interactions occur between the proteins. In particular, the side-chain amino group of T–TXNIP Arg251 forms a salt bridge with the side-chain carboxyl group of TRX Asp60, which further supports the interaction between TRX and T–TXNIP ( Fig. 3c ). Interestingly, this interaction pattern is similar to that of TRX complexed with NF-κB [37] and Ref-1 (ref. 38 ), which are implicated in TRX-mediated disulphide bond reduction of cellular substrates ( Supplementary Fig. S6 ). The intermolecular backbone–backbone interactions that stabilize the TRX–TXNIP complex are strictly conserved in both of these complexes. 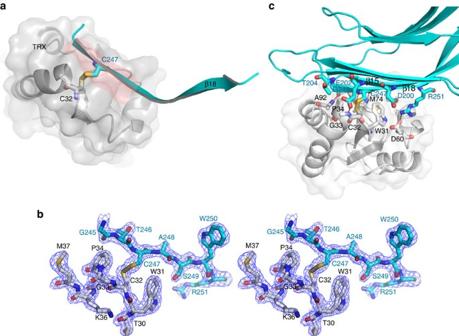Figure 3: Detailed characterization of the TRX–TXNIP interaction. (a) The critical β18 strand (cyan) of TXNIP that interacts with TRX is shown. The cleft formed by residues in the active site of TRX is highlighted in pink. The TRX Cys32 and TXNIP Cys247 residues that form an intermolecular disulphide bond are shown as white and cyan carbon atoms, respectively. (b) Stereo image of the 2Fo-Fc electron density map showing the intermolecular disulphide bond between the TRX Cys32 (white) and TXNIP Cys247 (cyan) residues contoured at 1.5σ. (c) Detailed depiction of the interactions between TRX (white) and TXNIP (cyan). The backbone–backbone interactions between TRX Met74 and TXNIP Cys247, and TRX Ala92 and TXNIP Gly245, are displayed as dashed red lines. The salt bridge between TRX Asp60 and TXNIP Arg251 and the hydrogen bond between TRX Gly33 and TXNIP Glu202 are shown as dashed black lines. Strands β15 and β18 in TXNIP are also indicated. Figure 3: Detailed characterization of the TRX–TXNIP interaction. ( a ) The critical β18 strand (cyan) of TXNIP that interacts with TRX is shown. The cleft formed by residues in the active site of TRX is highlighted in pink. The TRX Cys32 and TXNIP Cys247 residues that form an intermolecular disulphide bond are shown as white and cyan carbon atoms, respectively. ( b ) Stereo image of the 2Fo-Fc electron density map showing the intermolecular disulphide bond between the TRX Cys32 (white) and TXNIP Cys247 (cyan) residues contoured at 1.5σ. ( c ) Detailed depiction of the interactions between TRX (white) and TXNIP (cyan). The backbone–backbone interactions between TRX Met74 and TXNIP Cys247, and TRX Ala92 and TXNIP Gly245, are displayed as dashed red lines. The salt bridge between TRX Asp60 and TXNIP Arg251 and the hydrogen bond between TRX Gly33 and TXNIP Glu202 are shown as dashed black lines. Strands β15 and β18 in TXNIP are also indicated. Full size image TXNIP molecules form an interprotomer disulphide bond The TXNIP–TRX interaction requires oxidized TXNIP, which is thought to contain an intramolecular disulphide bond between Cys63 and Cys247, and reduced TRX [34] . However, the way in which the interaction forms is unknown. In the T–TXNIP structure, Cys63 is located 39 Å from Cys247 ( Fig. 2a ). Given this distance, intramolecular contact between the two residues is unlikely. Therefore, we hypothesized that Cys63 and Cys247 may form interprotomer disulphide bonds between TXNIP molecules. To test this hypothesis, the interaction between TXNIP molecules was examined using 293 T cells transfected with HA-tagged TXNIP and FLAG-tagged T–TXNIP. Lysis buffer containing iodoacetamide was used to avoid redox reactions during cell lysis, leading to non-specific disulphide bond formation. Immunoprecipitation experiments revealed an interprotomer interaction between TXNIP molecules ( Supplementary Fig. S7a ), and a high molecular weight T–TXNIP complex was detected dependent on the redox conditions ( Supplementary Fig. S7b ). Immunoblot analysis also demonstrated that TXNIP molecules interact with each other in vivo and that the N- and C-terminal domains are both required for the interaction ( Fig. 4a ). We specifically evaluated the roles of Cys63 in the N-terminal domain and Cys247 in the C-terminal domain using GST-fused and FLAG-tagged TXNIP. The introduction of C247S mutations into both of the tagged TXNIP proteins abolished the interaction, whereas the interaction was not affected when only the GST-fused TXNIP was mutated ( Fig. 4b ). The same results were obtained upon the introduction of C63S mutations ( Fig. 4b ). These results suggest that TXNIP molecules form a head-to-tail interprotomer disulphide bond between Cys63 and Cys247. 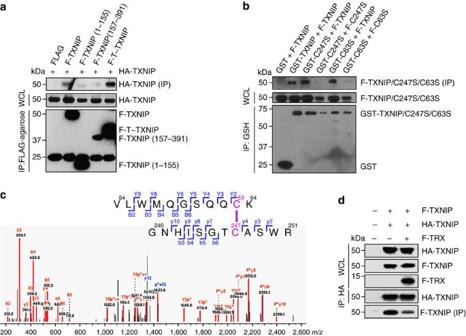Figure 4: TXNIP molecules form interprotomer disulphide bonds between Cys63 and Cys247. (a,b) Co-immunoprecipitation assays were performed using lysates from 293 T cells transfected with combinations of FLAG-tagged (F), HA-tagged, and GST-tagged full-length TXNIP, T–TXNIP, or mutant TXNIP. Immobilized proteins on FLAG-agarose beads or glutathione beads were visualized by immunoblotting using anti-HA, anti-FLAG, or anti-GST antibodies. One percent of the WCL was used as the input. (c) Proteomic analysis of the interprotomer-interacting TXNIP molecules fractionated by SDS–PAGE under non-reducing conditions. The MS/MS spectrum shows the interprotomer disulphide bond between Cys63 and Cys247 identified as54VLWMQGSQQCK64-240GNHISGTCASWR251. Doubly charged [M+2H]+peptide ions atm/z1353.64 were fragmented via higher-energy collisional dissociation. Matched peaks are shown in red. The ion types of matched peaks are written in red for b- and y-ions and blue for ions from C-S and S-S bond cleavages. Annotations used are: P, strand VLWMQGSQQCK; p, strand GNHISGTCASWR; B and Y, ions from P; b and y, ions from p; p+32, persulfide ion of p formed by C-S bond cleavage reactions. (d) The effect of TRX on the interaction between TXNIP molecules. Co-immunoprecipitation assays were performed using lysates from 293 T cells transfected with FLAG-tagged TXNIP, HA-tagged TXNIP and FLAG-tagged TRX. Immobilized proteins on HA-agarose beads were visualized by immunoblotting using anti-HA and anti-FLAG antibodies. (a,b,d) The results are representative of at least two independent experiments with similar results. Figure 4: TXNIP molecules form interprotomer disulphide bonds between Cys63 and Cys247. ( a , b ) Co-immunoprecipitation assays were performed using lysates from 293 T cells transfected with combinations of FLAG-tagged (F), HA-tagged, and GST-tagged full-length TXNIP, T–TXNIP, or mutant TXNIP. Immobilized proteins on FLAG-agarose beads or glutathione beads were visualized by immunoblotting using anti-HA, anti-FLAG, or anti-GST antibodies. One percent of the WCL was used as the input. ( c ) Proteomic analysis of the interprotomer-interacting TXNIP molecules fractionated by SDS–PAGE under non-reducing conditions. The MS/MS spectrum shows the interprotomer disulphide bond between Cys63 and Cys247 identified as 54 VLWMQGSQQ C K 64 - 240 GNHISGT C ASWR 251 . Doubly charged [M+2H] + peptide ions at m/z 1353.64 were fragmented via higher-energy collisional dissociation. Matched peaks are shown in red. The ion types of matched peaks are written in red for b- and y-ions and blue for ions from C-S and S-S bond cleavages. Annotations used are: P, strand VLWMQGSQQCK; p, strand GNHISGTCASWR; B and Y, ions from P; b and y, ions from p; p+32, persulfide ion of p formed by C-S bond cleavage reactions. ( d ) The effect of TRX on the interaction between TXNIP molecules. Co-immunoprecipitation assays were performed using lysates from 293 T cells transfected with FLAG-tagged TXNIP, HA-tagged TXNIP and FLAG-tagged TRX. Immobilized proteins on HA-agarose beads were visualized by immunoblotting using anti-HA and anti-FLAG antibodies. ( a , b , d ) The results are representative of at least two independent experiments with similar results. Full size image Mass spectrometry was employed to analyse the interprotomer disulphide bond between Cys63 and Cys247. The presence of other potential TXNIP-interacting cellular proteins or non-specific binding proteins made it difficult to isolate the interprotomer-interacting TXNIP molecules from 293 T cells transfected with plasmids expressing GST-fused TXNIP ( Supplementary Fig. S8 and Supplementary Tables S1 and S2 ). Therefore, the non-specific covalent oligomerization-preventing T–TXNIP(C36S/C49S/C120S/C170S/C205S/C267S) protein isolated from the TRX(C73A)–T–TXNIP(C36S/C49S/C120S/C170S/C205S/C267S) complex was used to induce interprotomer-interacting TXNIP molecules in vitro ( Supplementary Fig. S9a ), and the fractionated protein bands were subjected to mass spectrometric analysis. Protein bands of approximately 32 kDa and 60 kDa, which represented the monomeric T–TXNIP mutant and interprotomer-interacting protein complex, respectively, were identified by non-reducing SDS–PAGE ( Supplementary Fig. S9b ), and disulphide bonds with Dbond scores greater than 20 were identified at Cys63-Cys190, Cys63-Cys247, Cys63-Cys63, Cys190-Cys247 and Cys247-Cys247 ( Supplementary Fig. S9c ). However, the distribution of disulphide bond sites differed between the bands. In the 60 kDa band, Cys63-Cys247 was identified as the major disulphide bond, while Cys63-Cys190 was the major bond in the 32 kDa band ( Supplementary Table S3 ). Furthermore, the sites of free cysteines, which appeared as carbamidomethyl cysteines after alkylation, had different distributions in the two bands. A large number of free cysteines, particularly Cys190, were identified in the 32 kDa band ( Supplementary Table S3 ). Representative MS/MS spectra of the Cys63-Cys190 bond in the 32 kDa band and the Cys63-Cys247 bond in the 60 kDa band are shown in Supplementary Fig. S9c and Fig. 4c , respectively. Taken together, these data demonstrate that TXNIP molecules interact via a head-to-tail interprotomer disulphide bond between Cys63 and Cys247. On the other hand, size-exclusion experiments demonstrated that TRX-bound TXNIP exists predominantly in a heterodimeric form in solution ( Supplementary Fig. S2 ). To evaluate the effect of TRX on the interaction between TXNIP molecules, we performed co-immunoprecipitation assays using lysates of 293 T cells transfected with FLAG-tagged TXNIP, HA-tagged TXNIP, and FLAG-tagged TRX. The interaction between TXNIP molecules was markedly diminished by the overexpression of TRX ( Fig. 4d ). TRX–TXNIP interaction undergoes disulphide bond switching Although the results of co-immunoprecipitation and mass spectrometry studies indicated that a head-to-tail interprotomer disulphide bond between Cys63 and Cys247 of TXNIP molecules is involved in its interaction with TRX, it is noteworthy that TRX interacts exclusively with C-TXNIP. A possible explanation for this apparent contradiction is that Cys63 is involved in a transient interaction with TRX prior to the formation of the final TRX–TXNIP complex. Interestingly, we found that N-TXNIP (residues 3–156) was co-purified with TRX or TRX(C35A) ( Supplementary Fig. S10a ). To further evaluate the interaction of N-TXNIP with TRX, an NMR-titration was performed by recording a series of 1 H– 15 N heteronuclear single quantum coherence (HSQC) spectra of 15 N-labelled N-TXNIP after the addition of unlabelled reduced TRX. The addition of TRX caused substantial chemical shifts, indicating a direct interaction between N-TXNIP and TRX ( Supplementary Fig. S10b ). However, attempts to crystallize N-TXNIP and TRX(C35A) in complex were unsuccessful, suggesting that the interaction between the two proteins is transient. Because reduced TRX only binds to disulphide bonds [34] , we assumed that a disulphide bond is also involved in the interaction with N-TXNIP. To test this hypothesis, the structure of N-TXNIP was determined at 1.6 Å resolution ( Fig. 5a and Table 2 ). The structure obtained was generally similar to that of the corresponding domain in T–TXNIP. However, unlike T–TXNIP, an unexpected intramolecular disulphide bond between Cys63 and Cys120 was detected ( Fig. 5a ). In the structure, the distance between Cys63 and Cys120 is 14.1 Å ( Fig. 2a ), which is too large for the formation of a disulphide bond, and Cys120 is not involved in TRX binding [34] . Furthermore, alignment of the amino acid sequences of TXNIPs from four species showed that, while Cys63, Cys170, Cys190, Cys205, Cys247 and Cys267 are strictly conserved, Cys36, Cys49, Cys120, Cys333 and Cys384 are not ( Supplementary Fig. S11 ), providing further evidence that Cys120 is not essential for TRX binding. Therefore, the unexpected disulphide bond observed between Cys63 and Cys120 in N-TXNIP may be an artificial consequence, but it is likely that Cys63 requires another orphan cysteine residue (such as Cys247) to form a disulphide bond. N-TXNIP contains other cysteine residues at positions 36 and 49, which are located 49 Å and 22 Å from Cys63, respectively ( Fig. 5a ). These distances are too far to allow disulphide bond formation. Recently, Polekhina et al. [39] reported the two different crystal structures of N-TXNIP(C36S/C49S/K64A/C120S) and N-TXNIP(C36S/C49S/C120S) (residues 1–149) (ref. 39 ). Although the overall structures of these two N-TXNIP proteins and the N-TXNIP protein used here are very similar, significant conformational changes were detected in the β5 and Cys63-containing β6 strands ( Fig. 5b ). Interestingly, Polekhina et al. reported that the N-TXNIP(C36S/C49S/C120S) structure contains a Cys63-Cys63 intermolecular disulphide bond [39] that causes a conformational change of the β5 and β6 strands in crystallographically independent molecules ( Fig. 5b ). Taken together, these observations suggest that TXNIP undergoes a Cys63-mediated conformational change during its interaction with TRX. 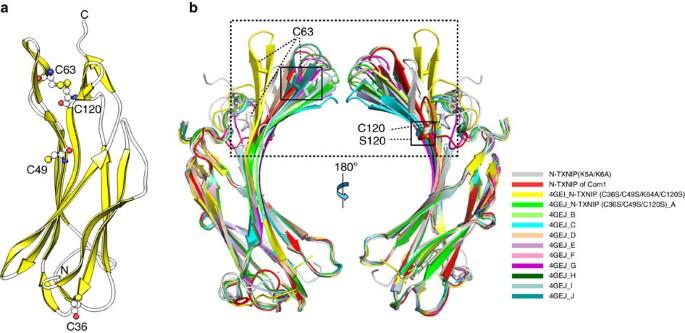Figure 5: N-TXNIP undergoes a Cys63-mediated conformational change. (a) Ribbon representation of N-TXNIP showing the intramolecular disulphide bond between Cys63 and Cys120. The locations of other cysteine residues are also shown. (b) N-TXNIP structures were superimposed onto the N-TXNIP(K5A/K6A) structure (grey). The structure of N-TXNIP(C36S/C49S/K64A/C120S) (Protein Data Bank accession code 4GEI) is shown in yellow. The structures of the crystallographically independent molecules of N-TXNIP(C36S/C49S/C120S) (Protein Data Bank accession code 4GEJ) are shown in different colours. The N-terminal domain of Com1 (red) has a similar conformation to the D-chain structure (wheat) of N-TXNIP(C36S/C49S/C120S). The region that undergoes significant structural changes between the N-TXNIP structures is indicated by the black dashed line box. The locations of the Cys63, Cys120 and Ser120 residues are indicated. Figure 5: N-TXNIP undergoes a Cys63-mediated conformational change. ( a ) Ribbon representation of N-TXNIP showing the intramolecular disulphide bond between Cys63 and Cys120. The locations of other cysteine residues are also shown. ( b ) N-TXNIP structures were superimposed onto the N-TXNIP(K5A/K6A) structure (grey). The structure of N-TXNIP(C36S/C49S/K64A/C120S) (Protein Data Bank accession code 4GEI) is shown in yellow. The structures of the crystallographically independent molecules of N-TXNIP(C36S/C49S/C120S) (Protein Data Bank accession code 4GEJ) are shown in different colours. The N-terminal domain of Com1 (red) has a similar conformation to the D-chain structure (wheat) of N-TXNIP(C36S/C49S/C120S). The region that undergoes significant structural changes between the N-TXNIP structures is indicated by the black dashed line box. The locations of the Cys63, Cys120 and Ser120 residues are indicated. Full size image Table 2 Data collection and refinement statistics for N-TXNIP structure. Full size table Superimposition of the T–TXNIP and N-TXNIP structures revealed that, compared with the corresponding region in T–TXNIP, formation of the disulphide bond between Cys63 and Cys120 in N-TXNIP causes a clockwise shift of approximately 96°, a 54° downward bending of strands β5 and β6, and a marked change in the β8 to β10 region ( Fig. 6a ). This movement leads to a change in the secondary structures of the β5 and β6 strands, which are critical for interdomain interactions between N-TXNIP and C-TXNIP in the TRX–TXNIP complex (see below). NMR 1 H– 15 N HSQC experiments performed using 15 N-labelled N-TXNIP mutants and TRX indicated a lack of chemical shifts in the spectra of either the C63S or C120S N-TXNIP mutants in the presence of TRX ( Supplementary Fig. S12 ). This result further corroborates the notion that the binding of TRX to TXNIP is initiated by a transient interaction between TRX and the interprotomer Cys63-Cys247 disulphide bond between TXNIP molecules. This transient interaction must result in the stable intermolecular interaction between TRX Cys32 and TXNIP Cys247 observed in the complex structure. Therefore, disruption of the interprotomer interaction between TXNIP molecules by TRX would leave Cys63 orphaned and reactive. T–TXNIP contains an interdomain disulphide bond between N-TXNIP Cys63 and C-TXNIP Cys190 ( Fig. 6a,b ), which suggests that the orphaned Cys63 immediately bonds to an available nearby cysteine to stabilize its state. The interaction between Cys63 and Cys190 causes the formation of a tight junction between the two domains, with the disulphide bond located in the centre of the interdomain interface, between the β-sheets of each domain ( Fig. 6b ). The disulphide bond is then surrounded by additional residues involved in the interface and is completely shielded from solvent. Therefore, the atypical S-shaped domain conformation of TXNIP can be attributed to this unique mutual disposition of the two domains, which is mainly due to the disulphide bond between Cys63 and Cys190. Disruption of this interdomain disulphide bond may lead to striking structural changes (see Fig. 2a ). Additional interdomain interactions between the N-terminal β6 strand and the β19 strand on the other side of the C-terminal β-sheets were also detected ( Fig. 6c ). The side-to-side interaction between the β-sheets of the two domains seems to confirm the S-shaped conformation. These interdomain interactions of TXNIP differ from those reported for other arrestin family proteins; in general, the domain interface of arrestin proteins merely contains clusters of buried polar interactions [35] , [40] , [41] . 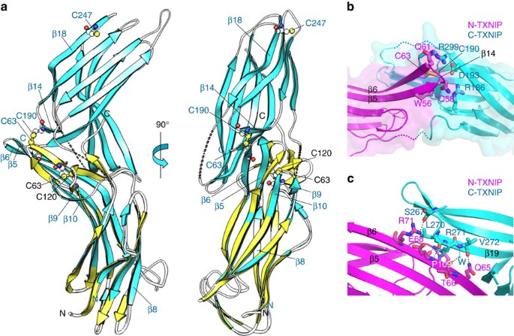Figure 6: The interaction between TRX and TXNIP involves disulphide bond switching. (a) TXNIP undergoes disulphide bond switching via a significant Cys63-mediated conformational change. The N-TXNIP structure (yellow) is superimposed onto the T–TXNIP structure (cyan). The interdomain disulphide bond between Cys63 and Cys190 in T–TXNIP and the intramolecular disulphide bond between Cys63 and Cys120 in N-TXNIP are indicated. (b) The interdomain disulphide bond formed between Cys63 of N-TXNIP (magenta) and Cys190 of C-TXNIP (cyan) is located at the centre of the interdomain interface. The residues involved in the interface are depicted using stick representations. The β5, β6, and β14 strands are also indicated. (c) A side-to-side interaction occurs between the TXNIP domains. The interdomain interactions between the N-terminal strand β6 (magenta) and the C-terminal strand β19 (cyan) are shown. Figure 6: The interaction between TRX and TXNIP involves disulphide bond switching. ( a ) TXNIP undergoes disulphide bond switching via a significant Cys63-mediated conformational change. The N-TXNIP structure (yellow) is superimposed onto the T–TXNIP structure (cyan). The interdomain disulphide bond between Cys63 and Cys190 in T–TXNIP and the intramolecular disulphide bond between Cys63 and Cys120 in N-TXNIP are indicated. ( b ) The interdomain disulphide bond formed between Cys63 of N-TXNIP (magenta) and Cys190 of C-TXNIP (cyan) is located at the centre of the interdomain interface. The residues involved in the interface are depicted using stick representations. The β5, β6, and β14 strands are also indicated. ( c ) A side-to-side interaction occurs between the TXNIP domains. The interdomain interactions between the N-terminal strand β6 (magenta) and the C-terminal strand β19 (cyan) are shown. Full size image Together with the structure of the TRX–T–TXNIP complex and the results of the co-immunoprecipitation assays and mass spectrometric analyses, the isolated N-TXNIP structure and NMR analyses suggest that TRX and TXNIP interact via a novel disulphide bond-switching mechanism that involves the replacement of a head-to-tail interprotomer TXNIP Cys63-TXNIP Cys247 disulphide bond with an interdomain TXNIP Cys63-Cys190 disulphide bond and a de novo intermolecular TXNIP Cys247-TRX Cys32 disulphide bond. ROS directly affect the TRX–TXNIP interaction The regulation of TRX by TXNIP is redox-dependent [34] , [42] . ROS activate the oxidative stress-responsive pathway and can alter protein structure and/or function [22] , [32] . Therefore, we examined the responsiveness of the TRX–T–TXNIP complex to ROS. To prevent non-functional cysteine-induced non-specific oligomerization of T–TXNIP and dimerization of TRX, experiments were performed using T–TXNIP(C120S/C170S/C205S/C267S) complexed with native TRX, or T–TXNIP(C36S/C49S/C120S/C170S/C205S/C267S) complexed with TRX(C73A), both of which contain intermolecular disulphide bonds between TXNIP Cys247 and TRX Cys32, and intramolecular disulphide bonds between TXNIP Cys63 and Cys190. Treatment of the TRX–T–TXNIP complex with H 2 O 2 or the thiol-oxidizing agent diamide resulted in dissociation of the proteins in a dose-dependent manner ( Fig. 7a,b ). The dissociated T–TXNIP was monomeric ( Fig. 7a,b ), indicating that ROS may react with the intermolecular disulphide bond between TRX Cys32 and TXNIP Cys247, while the TXNIP interdomain disulphide bond between Cys63 and Cys190 persists in oxidizing conditions. To confirm the role of Cys35 in the formation of the disulphide bond with Cys32 and dissociation from TXNIP under oxidizing conditions, the purified TRX(C35A) and T–TXNIP(C120S/C170S/C205S/C267S) complex was treated with 3.3 mM diamide. Unlike wild-type TRX, no dissociation of the proteins was observed ( Fig. 7c ). 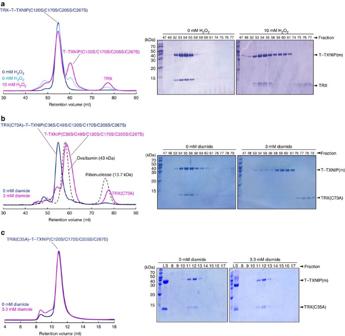Figure 7: ROS directly affect the intermolecular disulphide bond between TRX and TXNIP. (a,b) Size-exclusion chromatography analyses of the effect of ROS on the interaction between TRX and TXNIP. The TRX-T–TXNIP(C120S/C170S/C205S/C267S) complex was incubated with 0, 5, or 10 mM H2O2at 37 °C for 30 min (a) and the TRX(C73A)–T–TXNIP(C36S/C49S/C120S/C170S/C205S/C267S) complex was incubated with 0 or 3 mM diamide at 37 °C for 30 min (b). The reaction products were injected onto a HiLoad 16/60 Superdex 75 gel filtration column at room temperature. (c) The TRX(C35A)–T–TXNIP(C120S/C170S/C205S/C267S) complex was incubated with 3.3 mM diamide at 37 °C for 60 min. The reaction products were injected into a Superdex 75 10/300 GL gel filtration column at room temperature. (a–c) All eluted proteins were analysed by SDS–PAGE. T–TXNIP(m), T–TXNIP mutant; LS, loading solution. Figure 7: ROS directly affect the intermolecular disulphide bond between TRX and TXNIP. ( a , b ) Size-exclusion chromatography analyses of the effect of ROS on the interaction between TRX and TXNIP. The TRX-T–TXNIP(C120S/C170S/C205S/C267S) complex was incubated with 0, 5, or 10 mM H 2 O 2 at 37 °C for 30 min ( a ) and the TRX(C73A)–T–TXNIP(C36S/C49S/C120S/C170S/C205S/C267S) complex was incubated with 0 or 3 mM diamide at 37 °C for 30 min ( b ). The reaction products were injected onto a HiLoad 16/60 Superdex 75 gel filtration column at room temperature. ( c ) The TRX(C35A)–T–TXNIP(C120S/C170S/C205S/C267S) complex was incubated with 3.3 mM diamide at 37 °C for 60 min. The reaction products were injected into a Superdex 75 10/300 GL gel filtration column at room temperature. ( a – c ) All eluted proteins were analysed by SDS–PAGE. T–TXNIP(m), T–TXNIP mutant; LS, loading solution. Full size image Cellular redox homoeostasis is an essential defence mechanism against stimuli such as ROS and is crucial to a number of biological processes. TRX is involved in redox homoeostasis and regulates a wide range of cell signalling processes. Its endogenous inhibitor, TXNIP, modulates the redox system by binding to the active cysteine residue of TRX and inhibiting its antioxidative function [34] , [43] . The results presented here provide insight into the molecular basis of the negative regulation of TRX by TXNIP ( Fig. 8 ). Under normoxic conditions, TXNIP binds to TRX through an intermolecular disulphide bond and inhibits its reducing activity [32] . During oxidative stress, high levels of ROS may cause further oxidation of this bond, leading to the formation of thiosulfinates [44] . Such intermediates may react readily with any available thiol to form disulphide bonds, such as the bond between TRX Cys32 and Cys35, and sulfenic acid, such as TXNIP Cys247. As a consequence of these events, TXNIP dissociates from TRX. Unlike the wild-type complex, oxidative stress did not cause dissociation of the TRX(C35A)–TXNIP complex ( Fig. 7c ), suggesting that Cys35 is essential for the dissociation of the two proteins caused by targeting of the intermolecular disulphide between TRX Cys32 and TXNIP Cys247 by ROS. ROS also likely trigger antioxidant pathways that would then utilize the TRX system, including TRX reductase and NADPH, to restore a reducing environment. Reduction of the TXNIP interdomain disulphide bond between Cys63 and Cys190 would make Cys63 available to form an interprotomer disulphide linkage with Cys247 of another TXNIP molecule, as observed in in vivo co-immunoprecipitation and mass spectrometry experiments ( Fig. 4a–c ). After restoration of the reductive redox potential, the activity of TRX must be arrested. The active cysteines of TRX may then interact with the interprotomer disulphide bond between Cys63 and Cys247 of TXNIP molecules, which would perturb the interprotomer interaction and leave Cys63 orphaned and reactive. Subsequently, a large structural movement of the N-terminal domain of TXNIP would occur (particularly around strands β5 and β6), perhaps also involving the C-terminal domain ( Figs 5b and 6a ). Cys63 would then couple with C-terminal Cys190, producing close apposition of the domains and a different domain assembly (S-shape) to that of other arrestin family members (ω-shape). This unique fold would eventually facilitate the formation of a stable interaction interface mediated by an intermolecular disulphide bond between TXNIP Cys247 and TRX Cys32. This novel disulphide bond-switching mechanism provides a key insight into the TRX and TXNIP-dependent regulation of cell function, which is particularly important for understanding the pathophysiology of cancer and metabolic diseases. 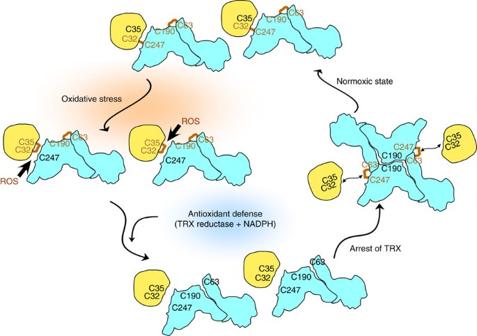Figure 8: Proposed molecular mechanism of the negative regulation of TRX by TXNIP. The inhibition of TRX by TXNIP is regulated by a redox-dependent disulphide bond-switching mechanism. Under normoxic conditions, TXNIP binds to TRX through an intermolecular disulphide bond formed between TXNIP Cys247 and TRX Cys32 and inhibits its reducing activity. During oxidative stress, high levels of ROS may cause further oxidation of this bond and lead to the dissociation of TXNIP from TRX. ROS also likely trigger antioxidant pathways to restore a reducing environment. After restoration of a reductive redox potential, the active cysteines of TRX may interact with the interprotomer disulphide bond between Cys63 and Cys247 of TXNIP molecules. Subsequently, TXNIP molecules would undergo a structural rearrangement that involves switching of the interprotomer disulphide bond between TXNIP molecules to an interdomain Cys63-Cys190 disulphide bond, and the formation of ade novointermolecular TXNIP Cys247-TRX Cys32 disulphide bond. See discussion for a full description. TRX and TXNIP are shown in yellow and cyan, respectively. Cysteine residues forming disulphide bonds are displayed in brown. Figure 8: Proposed molecular mechanism of the negative regulation of TRX by TXNIP. The inhibition of TRX by TXNIP is regulated by a redox-dependent disulphide bond-switching mechanism. Under normoxic conditions, TXNIP binds to TRX through an intermolecular disulphide bond formed between TXNIP Cys247 and TRX Cys32 and inhibits its reducing activity. During oxidative stress, high levels of ROS may cause further oxidation of this bond and lead to the dissociation of TXNIP from TRX. ROS also likely trigger antioxidant pathways to restore a reducing environment. After restoration of a reductive redox potential, the active cysteines of TRX may interact with the interprotomer disulphide bond between Cys63 and Cys247 of TXNIP molecules. Subsequently, TXNIP molecules would undergo a structural rearrangement that involves switching of the interprotomer disulphide bond between TXNIP molecules to an interdomain Cys63-Cys190 disulphide bond, and the formation of a de novo intermolecular TXNIP Cys247-TRX Cys32 disulphide bond. See discussion for a full description. TRX and TXNIP are shown in yellow and cyan, respectively. Cysteine residues forming disulphide bonds are displayed in brown. Full size image A recent study showed that the degradation of TXNIP is required for adipocyte differentiation and that overexpression of TRX prevents this process, thereby inhibiting adipogenesis [31] . TXNIP degradation mainly occurs via association of the E3 ubiquitin ligase Itch with the two PPxY motifs in the C-terminal region of TXNIP, leading to proteasomal degradation [45] . The authors speculated that the C-terminal tail of TXNIP may be tethered to the main body of the protein, thereby blocking Itch association. This proposed blocking mechanism is similar to that of β-arrestin, in which the C-terminal tail of the protein is tethered to the N-terminal arrestin domain, thereby blocking C-terminal tail-mediated protein–protein interactions [46] . The electron density map of T–TXNIP presented here was not visible beyond residue 299, suggesting the presence of a flexible region. Therefore, the C-terminal tail containing 331 PPxY 334 and 375 PPxY 378 would be connected to the flexible region ( Supplementary Fig. S13 ) [45] . An analysis of global ubiquitination in mammalian cells identified an ubiquitinated lysine at position 212 in TXNIP [47] . In the TXNIP–TRX complex, this residue is located in the highly basic C-terminal region, which forms a deeply curved β-sandwich domain that is inverted relative to N-TXNIP ( Supplementary Fig. S13 ). This location seems to be inaccessible to the E3 ubiquitin ligase Itch associated with the PPxY-containing C-terminal tail of TXNIP. Therefore, the increased stability of the TRX–TXNIP complex may be attributable to the exceptional S-shaped configuration of the protein, which may affect the ability of Itch to access the ubiquitination site rather than block the PPxY-containing C-terminal tail of TXNIP. On the other hand, the results presented here suggest that C-TXNIP is not properly folded, while N-TXNIP behaves as a globular protein. Accordingly, TRX-free TXNIP, including the TXNIP(C247S) mutant, should be flexible. Thus, its structure may not be S-shaped, which would allow Itch to access Lys212 and attach ubiquitin. We do not exclude the possibility that the inhibition of TRX by TXNIP is required to prevent adipogenesis. Adipogenesis is linked to oxidative stress [48] and Itch is known to regulate intracellular ROS levels [45] . TXNIP is a multifunctional protein that interacts with a variety of proteins involved in redox-independent cell signalling [42] . This feature may be characteristic of arrestin family members, which have emerged as molecular scaffolds and signal integrators. A recent review article suggested that, rather than functioning primarily as an inhibitor of TRX, TXNIP is an α-arrestin protein that is regulated by binding to TRX [49] , as occurs during adipogenesis [31] . Here, we demonstrated that TXNIP is a cysteine-containing redox protein that robustly regulates TRX via a novel disulphide bond-switching mechanism. This mechanism underlies a number of cell signalling pathways involved in cell growth, proliferation and metabolism. These properties are entirely distinct from other arrestin family members, including α- and β-arrestins [33] . In addition, the domain assembly of TXNIP differs from that of other arrestin proteins. Therefore, rather than classifying it as an arrestin protein, it may be prudent to describe TXNIP as a redox protein that contains an arrestin-like fold domain and functions in both a TRX-dependent and independent manner. TXNIP interacts with different cellular substrates using a variety of binding sites. For example, residues 1–227 of TXNIP interact with importin α1, leading to its nuclear localization [50] . In addition, the C-terminal region of TXNIP (residues 253–396) is critical for its interaction with JAB1 to stabilize p27(kip1) (ref. 51 ). These interactions do not involve TXNIP Cys247, suggesting a disulphide bond-switching-independent mechanism. Further experiments are required to confirm whether these binding partners can cause conformational changes and induce a general ω-shaped arrestin domain arrangement in TXNIP. DNA cloning and mutagenesis TXNIP could not be expressed as a soluble protein without TRX; therefore, plasmids co-expressing human TRX and TXNIP were constructed using a two-promoter vector system [52] . Briefly, the gene encoding T–TXNIP (residues 3–317) with an N-terminal hexahistidine-tag containing an integrated rTEV protease cleavage site was PCR amplified using the primers 5′-catgccatggtcaagaagatcaag-3′ and 5′-ataagaatgcggccgctcacattcagagctgg-3′ and cloned into the pProEX HTa plasmid (Invitrogen), which expresses tag-free human TRX under the control of the T7 promoter. A plasmid co-expressing human TRX and N-TXNIP (residues 3–156) was constructed using the same method with the primers 5′-ggaattccatatggtgaagcagat-3′ and 5′-ccgctcgagtcagactaattcattaat-3′ for human TRX, and primers 5′-catgccatggtcaagaagatcaag-3′ and 5′-ataagaatgcggccgctcataaatcagggg-3′ for N-TXNIP. N-TXNIP was also subcloned into the pHis-Parallel1 expression vector [53] , which includes an N-terminal hexahistidine-tag with an rTEV protease cleavage site. For NMR experiments, C-terminal hexahistidine-tagged TRX was subcloned into the pET21 vector (Invitrogen) using the primers 5′-ggaattccatatggtgaagcagat-3′ and 5′-ccgctcgaggactaattcattaat-3′. Mutations were introduced into the plasmids using the QuikChange Mutagenesis Kit (Stratagene), according to the manufacturer’s instructions. All constructs were verified by sequencing. Protein expression and purification Expression of wild-type and mutant TRX–T–TXNIP complexes and the TRX(C35A)–N-TXNIP complex was induced in Escherichia coli Rosetta gami (DE3) cells by treatment with 0.5 mM IPTG at 21 °C for 40 h. Expression of the N-TXNIP(K5A/K6A) mutant in E. coli C41(DE3) cells was induced by treatment with 0.5 mM IPTG at 21 °C for 16 h. Recombinant proteins were purified by Ni-NTA affinity chromatography, treated with rTEV protease to remove hexahistidine-tags, and then purified by size-exclusion chromatography and additional Ni-NTA affinity chromatography. The purified proteins were dialyzed against 50 mM Tris-HCl (pH 7.0). A selenomethionine (SeMet)-substituted complex of TRX(C35A) and T–TXNIP(C120S/C170S/C205S/C267S), and a SeMet-substituted N-TXNIP(K5A/K6A) complex, were expressed in the methionine auxotroph E. coli B834(DE3) strain (Novagen), which was grown in minimal medium supplemented with 50 mg ml −1 SeMet under the same conditions as cells containing the native plasmid. The SeMet-substituted proteins were purified as described for the native proteins. Expression of TRX was induced in E. coli C41 (DE3) cells by treatment with 0.5 mM IPTG at 21 °C for 18 h. The protein was purified by Ni-NTA agarose affinity and size-exclusion chromatography, and then dialyzed against 50 mM potassium phosphate (pH 6.6) for use in NMR experiments. E. coli C41 (DE3) cells transformed with plasmids encoding N-TXNIP or its mutants were grown in M9 minimal medium enriched with ( 15 NH 4 ) 2 SO 4 (99% 15 N) (Cambridge Isotope Laboratory Inc.) as the sole nitrogen source. All 15 N-labelled proteins were purified using Ni-NTA affinity chromatography. The proteins were treated with rTEV protease to remove the hexahistidine-tags and dialyzed against 50 mM potassium phosphate (pH 6.6) as the final step before NMR. Size-exclusion chromatography A Superdex 200 10/300 GL gel filtration column (GE Healthcare) installed on an AKTA purifier FPLC system (GE Healthcare) was equilibrated with 50 mM Tris-HCl (pH 8.0), 500 mM NaCl and 10% glycerol at a flow rate of 0.4 ml min −1 at room temperature. The purified TRX–T–TXNIP complex and its mutants were injected onto the column. Ovalbumin was used as the molecular weight standard. Crystallization and structure determination Because N-TXNIP was not crystallized, we crystallized an engineered derivative with reduced surface entropy [54] , N-TXNIP(K5A/K6A), using the sitting drop vapor-diffusion method at 21 °C. The best crystals were obtained with 0.75 M sodium-potassium phosphate and 0.1 M HEPES-Na (pH 7.5). Diffraction data were collected at beamline 4A (Pohang Accelerator Laboratory, Korea) at a resolution of 1.6 Å. SeMet-substituted K5A/K6A crystals were grown under the same conditions as the native protein. Multiple-wavelength anomalous diffraction data for the SeMet-substituted crystals were collected at beamline 6C at a resolution of 1.8 Å. The TRX(C35A) and T–TXNIP(C120S/C170S/C205S/C267S) complex crystals were optimized in 0.16 M tri-sodium citrate and 16% PEG 3350, and diffraction data were collected at a resolution of 2.0 Å at beamline 4A. SeMet-substituted crystals of the complex were grown in 0.2 M tri-sodium citrate and 20% PEG 3350. Multiple-wavelength anomalous diffraction data were collected at a resolution of 3.0 Å at beamline 6C. Crystals of the TRX(C35A) and T–TXNIP(C170S/C205S/C267S) complex were optimized using conditions similar to those used for the other complexes, and diffraction data were collected at a resolution of 2.7 Å at beamline 4A. All data were processed using the HKL2000 package [55] . The N-TXNIP(K5A/K6A) structure was determined by analysing anomalous signals from Se atoms with the program SOLVE [56] . Density modification and subsequent automated model building were performed using RESOLVE [57] . The native N-TXNIP(K5A/K6A) crystal structure was solved at a resolution of 1.6 Å using the MR method with the program MOLREP [58] , based on the partially refined structure of the SeMet crystal. The SeMet-substituted TRX(C35A) and T–TXNIP(C120S/C170S/C205S/C267S) structure was determined using SOLVE [56] , and subsequent automated model building was performed using RESOLVE [57] . The complex structure at a resolution of 2.0 Å was solved by MR using the partially refined SeMet complex structure. The TRX(C35A) and T–TXNIP(C170S/C205S/C267S) complex structure was determined by MR using the TRX(C35A) and T–TXNIP(C120S/C170S/C205S/C267S) complex model. All structures were revised using COOT [59] and refined with REFMAC5 (ref. 60 ). The crystallographic data are summarized in Tables 1 and 2 . Pull-down and co-immunoprecipitation assays To examine the in vivo interprotomer interaction between TXNIP molecules, HEK 293 T cells were transfected with plasmids expressing HA-tagged TXNIP and FLAG-tagged T–TXNIP. After 24 h, the cells were harvested and lysed in lysis buffer (0.5% Triton X-100, 150 mM NaCl, 10% glycerol, 1 mM NaF, 1 mM AEBSF, 2 μg ml −1 leupeptin, 5 μg ml −1 aprotinin and 20 mM HEPES (pH 7.2)) containing 50 mM iodoacetamide. After centrifugation at 16,000 × g for 20 min, the supernatant was incubated with anti-FLAG M2 agarose (Sigma) for 12 h at 4 °C. The agarose beads were collected by centrifugation and washed three times with lysis buffer. The bound proteins were then subjected to SDS–PAGE under reducing and non-reducing conditions. For the assay demonstrating the TXNIP–TXNIP interaction in detail, HEK 293 T cells were transfected with combinations of expression plasmids, as indicated in the main text. After 24 h, the cells were harvested, lysed and centrifuged at 16,000 × g for 20 min. The supernatants were incubated for 12 h at 4 °C with mouse monoclonal anti-FLAG M2 agarose beads (Sigma) for immunoprecipitation, or with glutathione-conjugated sepharose beads (GE Healthcare) for pull-down assays. The immobilized proteins were collected by centrifugation and washed three times with lysis buffer. Bound proteins or whole cell lysates (WCLs) were eluted by boiling in SDS sample buffer. To detect HA-tagged, FLAG-tagged or GST-fused proteins, rabbit polyclonal anti-HA (1:2,000), anti-FLAG (1:2,000) and anti-GST (1:1,000) antibodies (Santa Cruz Biotechnology) were used, respectively. Horseradish peroxidase-conjugated secondary antibody (1:5,000; Santa Cruz Biotechnology) was used to visualize the specific target bands. For the immunoprecipitation assay showing the effect of TRX on the TXNIP–TXNIP interaction, transfected HEK 293 T cells were harvested and lysed in buffer containing 0.5% Triton X-100, 150 mM NaCl, 10% glycerol, 20 mM HEPES (pH 7.2) and complete protease inhibitor cocktail (Roche). After incubation at 4 °C for 30 min, the lysate was centrifuged at 16,000 × g for 20 min. The supernatants were pre-cleared by incubation with 20 μl of protein G-sepharose beads (GE Healthcare) for 2 h at 4 °C, and then centrifuged at 10,000 × g for 5 min. The pre-cleared lysate was incubated for 14 h at 4 °C with the rabbit polyclonal anti-HA antibody, followed by 5 h at 4 °C with protein G-sepharose beads. After immunoprecipitation, the beads were washed five times with lysis buffer. Bound proteins or WCLs were eluted by boiling in LDS–PAGE loading buffer (Life Technologies). To detect HA-tagged proteins or FLAG-tagged proteins, a mouse monoclonal anti-HA antibody (1:2,000; Abcam) or anti-FLAG antibody (1:2,000; Sigma) was used, and then horseradish peroxidase-conjugated secondary antibody (1:5,000) or peroxidase-conjugated light chain-specific secondary antibody (1:3,500; Jackson ImmunoResearch Laboratories Inc.) was used to visualize the specific target bands. TRX activity assay TRX activity was measured using the insulin disulphide reduction assay, as described previously [10] . Briefly, HEK 293 T cells were mock-transfected or transiently transfected with TXNIP or mutant TXNIP expression plasmids. The transfected cells were lysed in buffer containing 20 mM HEPES (pH 7.9), 100 mM KCl, 300 mM NaCl, 10 mM EDTA, 0.1% Nonidet P-40 and protease inhibitors. To reduce TRX, cell extracts (20 μg) were incubated for 20 min at 37 °C with 2 μl of DTT activation buffer containing 1 mM EDTA, 1 mg ml −1 BSA, 2 mM DTT and 50 mM HEPES (pH 7.6) in a total volume of 70 μl. A 40 μl aliquot of reaction mixture taken from a solution containing 200 μl of 1 M HEPES (pH 7.6), 40 μl of 0.2 M EDTA, 40 μl of NADPH (40 mg ml −1 ) and 500 μl of insulin (10 mg ml −1 ) was then added. The reaction was started by the addition of 10 μl of rat TRX reductase (100 U ml −1 ) and incubated for 20 min at 37 °C. The reaction was stopped by the addition of 6 M guanidine-HCl and 1 mM DNTB (3-carboxy-4-nitrophenyl disulphide), and the absorbance at 412 nm was measured. Sample preparation for mass spectrometry For analysis by mass spectrometry in vivo , HEK 293 T cells were transfected with a plasmid expressing GST-fused TXNIP. After 24 h, the cells were harvested and lysed in buffer containing 0.5% Triton X-100, 150 mM NaCl, 10% glycerol, 20 mM HEPES (pH 7.2) and complete protease inhibitor cocktail. After incubation for 30 min at 4 °C, the lysates were centrifuged at 16,000 × g for 20 min. The supernatants were incubated overnight at 4 °C with Glutathione Sepharose 4FF (GE Healthcare) and then centrifuged at 10,000 × g for 5 min. The supernatant was discarded and the resin was washed five times with lysis buffer. Bound proteins were eluted by boiling in LDS–PAGE loading buffer. For analysis by mass spectrometry in vitro , the purified TRX(C73A)–T–TXNIP(C36S/C49S/C120S/C170S/C205S/C267S) complex was incubated with 100 mM DTT for 1 h at room temperature and then injected into a Superdex 200 10/300 GL gel filtration column installed on an AKTA purifier FPLC system to obtain T–TXNIP(C36S/C49S/C120S/C170S/C205S/C267S) and TRX(C73A). The fractions containing T–TXNIP(C36S/C49S/C120S/C170S/C205S/C267S) were dialyzed against 50 mM Tris-HCl (pH 8.0), 500 mM NaCl and 10% glycerol to induce the formation of disulphide bonds between TXNIP molecules through air oxidation. Dialyzed proteins were then subjected to non-reducing SDS–PAGE. In-gel digestion The high molecular weight TXNIP complex-containing gel pieces were destained in 25 mM ammonium bicarbonate and 50% acetonitrile, dehydrated with 100% acetonitrile and then dried at room temperature. Free cysteines were alkylated by adding 55 mM iodoacetamide in 25 mM ammonium bicarbonate and then incubated for 1 h at 25 °C in the dark. The gel was washed three times with 25 mM ammonium bicarbonate and 50% acetonitrile solution, dehydrated with 100% acetonitrile and then dried at room temperature. The gel pieces were rehydrated with a solution of 12.5 ng μl −1 sequencing-grade trypsin (Promega) in 25 mM ammonium bicarbonate and incubated for 16 h at 37 °C for protein digestion. The supernatants were transferred to fresh tubes and the remaining peptides were sequentially extracted by incubating the gel pieces with 50% acetonitrile in 25 mM ammonium bicarbonate, 50% acetonitrile in 0.5% trifluoroacetic acid and then 70% acetonitrile in 0.5% trifluoroacetic acid. The extracted peptides were combined, dried in a miVac Duo vacuum evaporator (Genevac) and stored at −20 °C until use [61] . Mass spectrometry The peptides were diluted with 0.4% acetic acid to achieve concentrations of 1 μg μl −1 and an aliquot containing approximately 1 μg was injected into a reversed-phase Magic C18aq column (15 cm × 75 μm) on an Eksigent nanoLC-ultra 1D plus system at a flow rate of 300 nl min −1 . Prior to use, the column was equilibrated with 95% buffer A (0.1% formic acid in H 2 O) and 5% buffer B (0.1% formic acid in acetonitrile). The peptides were eluted with a linear gradient from 10% buffer B to 40% buffer B over 40 min. The HPLC system was coupled to a Q Exactive quadrupole mass spectrometer (Thermo Scientific) operated in the data dependent mode. Survey full-scan MS spectra ( m/z 300–2000) were acquired in the Orbitrap with a resolution of 75,000. The MS/MS spectra of the 12 most intense ions from the MS1 scan with a charge state ≥2 were acquired with the following options: resolution, 17,500; isolation width, 2 m / z ; normalized collision energy, 27%; dynamic exclusion duration, 30 s; and ion selection threshold, 4.00E+03 counts. Database searching and validation The acquired MS/MS spectra were searched against the SwissProt database (August 2011) with 56,392 entries using X!Tandem open source software (available from http://www.thegpm.org/TANDEM/ ). The precursor mass tolerance was set to±15 p.p.m. and the cleavage specificity was set to trypsin, allowing for a maximum of one missed cleavage. A variable modification of methionine oxidation (+15.9949 Da) and carbamidomethylated cysteine (+57.0215 Da) was allowed. Peptide assignment was performed using the Trans Proteomics Pipeline (version 4.5 RAPTURE rev 2) provided by the Institute for Systems Biology ( http://www.proteomecenter.org ). From the X!Tandem search output, peptides with probabilities greater than 0.9 were included in the subsequent Protein-Prophet, and proteins with probabilities greater than 0.9 were gathered. Contaminants, such as keratin and trypsin artifacts, were removed from the results. The identification of disulphide linkages was performed using DBond software (version 3.02; http://prix.hanyang.ac.kr/download/dbond.jsp ) [62] . NMR spectroscopy NMR interaction experiments were performed by recording 1 H– 15 N NMR HSQC spectra of 15 N-labelled N-TXNIP, or its mutants, upon the addition of unlabelled TRX. Prior to the interaction study, TRX was reduced with 5 mM DTT and dialyzed against 50 mM potassium phosphate (pH 6.6) to remove excess DTT. The 1 H– 15 N HSQC spectra of all proteins were measured on a Bruker 900 MHz NMR spectrometer at the Korea Basic Science Institute (Ochang, Korea). The NMR measurements were performed in 50 mM potassium phosphate (pH 6.6) containing 10% D 2 O at 25 °C. All NMR spectra were processed with Topspin 2.1 and analysed with the program SPARKY 3.1. Analysis of the effect of ROS on the TRX–TXNIP interaction The TRX and T–TXNIP(C120S/C170S/C205S/C267S) complex was used to circumvent non-functional cysteine-induced aggregation. The complex (0.05 mM) was incubated at 37 °C with 0–10 mM H 2 O 2 in 50 mM Tris-HCl (pH 8.0), 500 mM NaCl and 10% glycerol. The TRX(C73A) and T–TXNIP(C36S/C49S/C120S/C170S/C205S/C267S) complex was also used to avoid TRX dimerization and non-functional cysteine-induced aggregation. This complex was incubated with 0–3 mM diamide in the same buffer at 37 °C. After 30 min, the samples were injected onto a HiLoad 16/60 Superdex 75 gel filtration column (GE Healthcare) installed on an AKTA purifier FPLC system at a flow rate of 1 ml min −1 at room temperature. To examine the role of TRX Cys35 in the dissociation of TRX and TXNIP, the TRX(C35A)–T–TXNIP(C120S/C170S/C205S/C267S) complex was incubated for 1 h at room temperature with 3.3 mM diamide and then injected into a Superdex 75 10/300 GL gel filtration column. All fractions were subjected to SDS–PAGE. Accession codes: The atomic coordinates and structure factor amplitudes of N-TXNIP, Com1, and Com2 have been deposited in the Protein Data Bank under accession codes 4GFX , 4LL1 and 4LL4 , respectively. How to cite this article: Hwang, J. et al. The structural basis for the negative regulation of thioredoxin by thioredoxin-interacting protein. Nat. Commun. 5:2958 doi: 10.1038/ncomms3958 (2014).